Three-layered polyplex micelle as a multifunctional nanocarrier platform for light-induced systemic gene transfer Nanocarriers responding to light have great potential for pinpoint therapy, and recent studies have revealed promising in vivo activity. However, light-selective gene transfer still remains challenging in the systemic application. Here we report systemic light-responsive nanocarriers for gene delivery developed through the sequential self-assembly of ABC-type triblock copolymer/DNA/dendrimeric photosensitizer, forming polyplex micelles with three-layered functional nanocompartments. The DNA-packaged core is covered by the photosensitizer-incorporated intermediate layer, which is encompassed by an outer shielding shell. This three-layered structure permits multistep photosensitizer and DNA delivery into a solid tumour by a systemic route: the shielding layer minimizes unfavourable interactions with blood components, and the photosensitizer is delivered to endo-/lysosomal membranes to facilitate light-selective cytoplasmic translocation of the micelles, accomplishing DNA delivery into the nucleus to exert gene expression. The polyplex micelles display >100-fold photoenhanced gene expression in cultured cells and exhibit light-induced in vivo gene transfer in solid tumours following systemic administration. Nanocarriers are aimed at delivering bioactive substances to target sites and eliciting their biological functions in a spatiotemporally controlled manner, thereby achieving enhanced therapeutic efficacy with minimal side effects [1] , [2] , [3] , [4] , [5] . These carriers need to achieve selective extravasation at target tissues after systemic administration, and a mechanism to circumvent intracellular barriers, such as effective transport from endosomal compartments to the cytoplasm, is indispensable for efficacy, particularly for gene and oligonucleotide delivery [6] . Physical energy in the form of light, ultrasound or magnetism can be used as a spatiotemporally controllable trigger to facilitate the overcoming of such biological barriers by nanocarriers [7] , [8] , [9] . Owing to recent advances in laser technology, light has become a useful and safe energy source, and laser therapy and photodynamic therapy are in practical use [10] , [11] , [12] . More recently, enhanced cytoplasmic delivery of macromolecular compounds by photochemical disruption of the endo-/lysosomal membrane, termed photochemical internalization (PCI), has attracted much attention [13] , [14] , [15] , [16] . Although PCI has been proven to work for gene transduction in cultured cells and epithelial tissues by local administration, this concept has yet to succeed in vivo in systemic applications. The greatest challenge in systemic PCI-mediated gene transduction is the simultaneous delivery of the gene (plasmid DNA; pDNA) and the photosensitizer (PS) to the target cell. Hence, nanocarriers need to incorporate both the pDNA and the PS; however, these molecules should be compartmentalized because a PS may inactivate pDNA through the formation of reactive oxygen species (ROS). In addition, nanocarriers should possess a shielding surface to avoid undesirable interactions with biological components. Here we report the first success in in vivo PCI-mediated gene transduction by systemic administration of a multi-compartmentalized nanocarrier newly designed for this purpose, as shown in Fig. 1 . The key to forming spatially segregated, three-layered compartments within a single nanocarrier platform is the sequential self-assembly of pDNA and dendrimeric PS (DPc) with triblock copolymers composed of tandemly aligned segments with distinct functionality in an aqueous solution. The nanocarrier thus has a core compartment for stable packaging of pDNA, an intermediate compartment for incorporation of DPc to induce PCI, and an outer hydrophilic compartment of poly(ethylene glycol) (PEG) that forms a shielding surface. The three-layered nanocarrier, termed DPc-TPM (a DPc-loaded ternary polyplex micelle), accommodates DPc and pDNA in these segregated compartments, thereby preventing photochemical damage to the encapsulated pDNA. Furthermore, integrated carboxylate groups on the periphery of the DPc contribute to its stable disposition in the intermediate cationic compartment. In turn, the acidic compartment of the endo-/lysosome neutralizes these carboxylate groups to facilitate the translocation of the amphiphilic DPc from the micellar compartment into the endo-/lysosomal membrane, thereby inducing a strong PCI effect. Consequently, using this DPc-TPM, successful PCI-mediated gene transduction through the systemic route is demonstrated in a xenografted tumour model in mice. 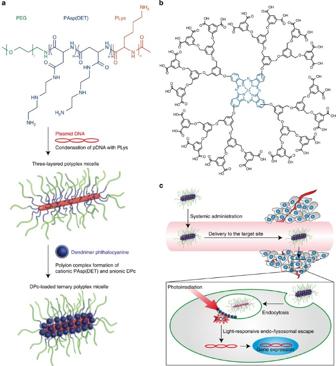Figure 1: Construction of the DPc-TPM and light-responsive gene transfer. (a) Design of the DPc-TPM. First, a three-layered polyplex micelle is prepared by mixing PEG-PAsp(DET)-PLys triblock copolymer and pDNA; the polyplex micelle is composed of a PEG shell, an intermediate PAsp(DET) layer and a PLys/pDNA core. The DPc-TPM is constructed by adding DPc to the PAsp(DET) intermediate layer. (b) Chemical structure of DPc. (c) Scheme showing the delivery at systemic and intracellular levels. At the systemic level, DPc-TPM circulates in the bloodstream; non-specific interaction with biological components is prevented after intravenous injection. In the target tissue (a solid tumour), DPc-TPMs are taken up by cells via endocytosis and entrapped in endo-/lysosomes. In response to the low pH prevalent in the endo-/lysosome, DPc is released from the DPc-TPMs owing to the protonation of the peripheral carboxyl groups and interacts with the endo-/lysosomal membrane through hydrophobic interactions. Upon photoirradiation, DPc generates ROS that destabilize the endo-/lysosomal membrane, facilitating endo-/lysosomal escape. Figure 1: Construction of the DPc-TPM and light-responsive gene transfer. ( a ) Design of the DPc-TPM. First, a three-layered polyplex micelle is prepared by mixing PEG-PAsp(DET)-PLys triblock copolymer and pDNA; the polyplex micelle is composed of a PEG shell, an intermediate PAsp(DET) layer and a PLys/pDNA core. The DPc-TPM is constructed by adding DPc to the PAsp(DET) intermediate layer. ( b ) Chemical structure of DPc. ( c ) Scheme showing the delivery at systemic and intracellular levels. At the systemic level, DPc-TPM circulates in the bloodstream; non-specific interaction with biological components is prevented after intravenous injection. In the target tissue (a solid tumour), DPc-TPMs are taken up by cells via endocytosis and entrapped in endo-/lysosomes. In response to the low pH prevalent in the endo-/lysosome, DPc is released from the DPc-TPMs owing to the protonation of the peripheral carboxyl groups and interacts with the endo-/lysosomal membrane through hydrophobic interactions. Upon photoirradiation, DPc generates ROS that destabilize the endo-/lysosomal membrane, facilitating endo-/lysosomal escape. Full size image Construction and characterization of DPc-TPMs First, pDNA and PEG-poly{ N -[ N -(2-aminoethyl)-2-aminoethyl]aspartamide}-poly(L-lysine) (PEG-PAsp(DET)-PLys; PEG: 12,000 (g mol −1 ), degree of polymerization (DP) of PAsp(DET): 34, DP of PLys: 52) were mixed at the stoichiometric charge ratio of PLys and pDNA ((amino groups in PLys)/(phosphate groups in pDNA); Lys/pDNA=1) to form pDNA/PEG-PAsp(DET)-PLys polyplex micelles. PLys has higher binding affinity to pDNA than PAsp(DET) [17] , [18] ; therefore, the PLys segment in the block copolymer selectively interacts with pDNA under this condition to form the three-layered polyplex micelle consisting of a PLys/pDNA polyplex core, a PAsp(DET) intermediate compartment and a PEG shell, as confirmed by 1 H NMR (proton nuclear magnetic resonance) measurement ( Supplementary Fig. 1 ). DPc with 32 carboxyl groups at the periphery (see the DPc chemical structure and absorption spectrum presented in Fig. 1b and Supplementary Fig. 2 , respectively) was then incorporated into the PAsp(DET) intermediate compartment through electrostatic interaction to create DPc-TPM for light-selective transfection. DPc was integrated into the three-layered polyplex micelles by simple mixing at various molar ratios of peripheral carboxyl groups on DPc to the protonated amino groups on PAsp(DET) (DPc/Asp(DET) ratios). Note that the side-chain diaminoethane units of PAsp(DET) are not completely protonated at pH 7.3 (these units are approximately in the single protonated state, according to a previously reported titration result) [19] . The simultaneous incorporation of pDNA and DPc into the micelles was confirmed by gel retardation assay and ultracentrifugation ( Supplementary Figs 3 and 4 ). The gel retardation assay revealed complete pDNA incorporation into the micelle at the DPc/Asp(DET) ratio of 0–4 ( Supplementary Fig. 3 ). At DPc/Asp(DET) ratios >4.5, appreciable release of pDNA from the micelles was observed, suggesting the replacement of pDNA by excess DPc. The ultracentrifugation study provided quantitative information on micelle composition ( Supplementary Fig. 4 ). At the DPc/Asp(DET) ratio of 1 (charge stoichiometric ratio), almost all DPc (98%) was incorporated into micelles. Interestingly, the proportional incorporation of DPc into micelles was observed even under an excess charge ratio of DPc to PAsp(DET) (DPc/Asp(DET) ratio of 2–4). Because DPc is known to induce secondary aggregation at higher concentrations in aqueous solution owing to hydrophobic interactions, even at pH 7.4 (ref. 20 ), DPc deposited within the PAsp(DET) compartment may facilitate further inclusion of DPc molecules above the stoichiometric charge ratio. Indeed, as the DPc/Asp(DET) ratio increased over the charge stoichiometry, the zeta potentials of the micelles were accordingly shifted to negative values ( Supplementary Fig. 5 ), which is consistent with DPc inclusion beyond the charge stoichiometry. The size and morphology of the three-layered polyplex micelles and the DPc-TPM were evaluated by transmission electron microscopy (TEM) after pDNA staining with uranyl acetate ( Fig. 2a–d ). The polyplex micelles (without DPc) exhibited characteristic rod-shaped structures ( Fig. 2a ). We also observed micelle shrinkage with a significant decrease in the major rod axis length through complex formation with DPc at a DPc/Asp(DET) ratio of 1 ( Fig. 2b and e ). The major rod axis length increased with further increases in the DPc/Asp(DET) ratio to 2 and 3 ( Fig. 2c–e ) as illustrated in Fig. 2f . This tendency towards morphological change was consistent with dynamic light scattering measurements ( Supplementary Figs 6–8 ), which showed a smaller cumulant diameter and a lower polydispersity index at the DPc/Asp(DET) ratio of 1. 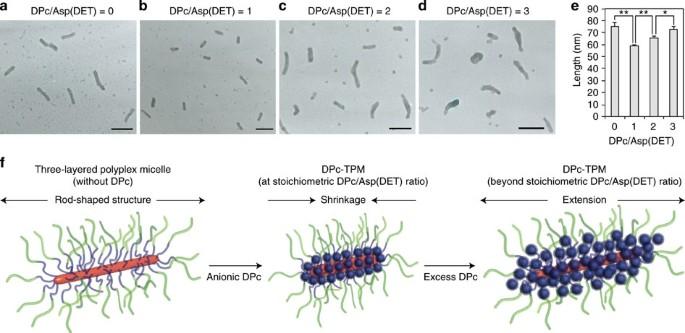Figure 2: TEM images of three-layered polyplex micelles and DPc-TPMs. (a–d) The morphology of the three-layered polyplex micelles and the DPc-TPMs was observed using TEM at 50,000-fold magnification: (a) pDNA/PEG-PAsp(DET)-PLys polyplex micelles (DPc/Asp(DET)=0); (b–d) DPc-TPMs (DPc/Asp(DET)=1–3). pDNA was visualized by staining with uranyl acetate. Scale bars, 100 nm. (e) The major axis length of the packaged pDNA within the polyplex micelles was measured based on the TEM images. The results are expressed as means±s.e.m. (n=100). *P<0.05, **P<0.01 (t-test). (f) A schematic diagram used to explain the results shown ina–e. Figure 2: TEM images of three-layered polyplex micelles and DPc-TPMs. ( a – d ) The morphology of the three-layered polyplex micelles and the DPc-TPMs was observed using TEM at 50,000-fold magnification: ( a ) pDNA/PEG-PAsp(DET)-PLys polyplex micelles (DPc/Asp(DET)=0); ( b – d ) DPc-TPMs (DPc/Asp(DET)=1–3). pDNA was visualized by staining with uranyl acetate. Scale bars, 100 nm. ( e ) The major axis length of the packaged pDNA within the polyplex micelles was measured based on the TEM images. The results are expressed as means±s.e.m. ( n =100). * P <0.05, ** P <0.01 ( t -test). ( f ) A schematic diagram used to explain the results shown in a – e . Full size image To gain further insight into the physicochemical properties of the DPc-TPM, the condensation level of pDNA in the polyplex was estimated by fluorescence resonance energy transfer (FRET). Here, pDNA was simultaneously labelled with fluorescein and Cy3. In the free form, fluorescein-Cy3-labelled pDNA emits efficient fluorescein fluorescence when excited at 470±10 nm. Upon pDNA condensation by a polycation, fluorescein-Cy3-labelled pDNA emits Cy3 fluorescence owing to FRET between fluorescein and Cy3. Hence, FRET efficiency indicates the pDNA condensation state [21] , [22] . We measured the FRET efficiency of DPc-TPM using different amounts of fed DPc. We also examined FRET efficiency in two other polyplexes as controls. One control was a randomly mixed TPM (random-TPM), which was prepared by randomly mixing pDNA, DPc and PEG-PAsp(DET)-PLys. The other control was a TPM without the intermediate layer (diblock-TPM), which was prepared by adding DPc to a pDNA/PEG-PLys polyplex micelle (PEG: 12,000 (g mol −1 ), DP of PLys: 45, Lys/pDNA=1.5) having no intermediate compartment. The preparation of these polyplexes is illustrated in Fig. 3a–c . FRET efficiency was defined as the ratio of fluorescein intensity to Cy3 fluorescence intensity (fluorescein/Cy3) and is summarized in Fig. 3d . In the absence of DPc, all micelles exhibited similar fluorescein/Cy3, indicating similar states of pDNA condensation. For the two control samples, an increase in DPc concentration led to marked enhancement in fluorescein/Cy3, indicating decreased FRET efficiency. This result is reasonably explained by a scheme in which DPc interaction attenuates pDNA condensation. By contrast, the DPc-TPMs did not exhibit any increase in fluorescein/Cy3 from the original value. This result is consistent with the three-layered structure of the DPc-TPM in which pDNA is well segregated from the PAsp(DET) layer through selective complexation with PLys, eventually maintaining the integrity of the condensed state even in the presence of anionically charged DPc. 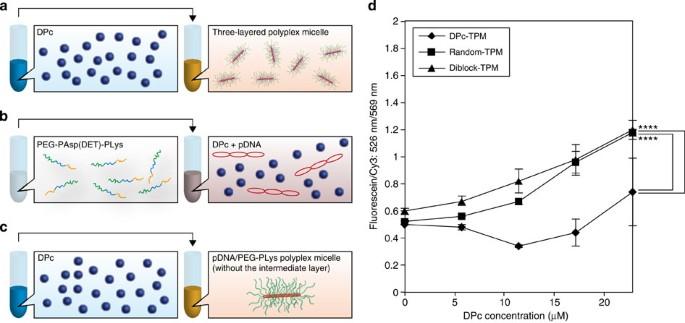Figure 3: The effect of DPc concentration on pDNA condensation. (a–c) The preparation of (a) DPc-TPMs, (b) random-TPMs, and (c) diblock-TPMs. (d) FRET induced by the condensation of pDNA labelled with fluorescein and Cy3. Fluorescein/Cy3 (fluorescence intensity at 526 nm/fluorescence intensity at 569 nm) of DPc-TPMs, random-TPMs and diblock-TPMs was calculated as a FRET indicator and plotted against DPc concentration. The DPc concentration of 5.7 μM is equivalent to a DPc/Asp(DET) ratio of 1 in DPc-TPMs. The results are expressed as means±s.e.m. (n=3). ****P<0.0001 (two-way analysis of variance using the Tukey–Kramer test). Figure 3: The effect of DPc concentration on pDNA condensation. ( a – c ) The preparation of ( a ) DPc-TPMs, ( b ) random-TPMs, and ( c ) diblock-TPMs. ( d ) FRET induced by the condensation of pDNA labelled with fluorescein and Cy3. Fluorescein/Cy3 (fluorescence intensity at 526 nm/fluorescence intensity at 569 nm) of DPc-TPMs, random-TPMs and diblock-TPMs was calculated as a FRET indicator and plotted against DPc concentration. The DPc concentration of 5.7 μM is equivalent to a DPc/Asp(DET) ratio of 1 in DPc-TPMs. The results are expressed as means±s.e.m. ( n =3). **** P <0.0001 (two-way analysis of variance using the Tukey–Kramer test). Full size image ROS generated by photoirradiated PS may damage nearby pDNA. We assume that compartmentalizing and segregating pDNA and DPc in the DPc-TPM reduces photochemical damage to pDNA. In this study, we photoirradiated DPc-TPMs (DPc/Asp(DET)=2) and random-TPMs (DPc/Asp(DET)=2) using a 300-W halogen lamp (fluence rate, 3.0 mW cm −2 ) equipped with a band filter (400–700 nm) and then quantified the amount of intact pDNA using electrophoresis ( Supplementary Fig. 9 ). Without photoirradiation, pDNA remained intact in both cases as confirmed based on the SYBR Green I fluorescence intensities of supercoiled pDNA. Smeared pDNA bands were evident in both cases with photoirradiation. However, a higher fraction of intact supercoiled pDNA was observed in DPc-TPMs (69% and 49% of the original fluorescence intensity after photoirradiation with 2 J cm −2 and 4 J cm −2 , respectively) compared with that in random-TPMs (51% and 27% of the original fluorescence intensity after photoirradiation with 2 J cm −2 and 4 J cm −2 , respectively, under the same conditions). This result strongly suggests that the pDNA condensed in the inner core was successfully compartmentalized and segregated from the DPc-incorporated intermediate layer, thereby allowing pDNA to avoid oxidative damage by ROS produced by DPc. In vitro activity of DPc-TPMs The internalization of DPc-TPMs into HeLa cells (cancerous cells) and HUVECs (human umbilical vein endothelial cells; normal cells) was evaluated using confocal laser scanning microscopy (CLSM) ( Supplementary Fig. 10 and Supplementary Methods ). Although the DPc-TPMs were internalized into both HeLa cells and HUVECs ( Supplementary Fig. 10a,b ), significantly higher cellular uptake was observed in HeLa cells than in HUVECs ( Supplementary Fig. 10e ). It is known that cancerous cells take up more circumjacent substances than normal cells, accounting for the difference in the cellular uptake. Following cellular internalization, DPc-TPMs are expected to release DPc under acidic conditions in the endo-/lysosomes because the peripheral carboxyl groups of DPc undergo protonation at pH 5.5 (ref. 23 ). Simultaneously, DPc exhibiting increased hydrophobicity because of the protonation of peripheral carboxyl groups may interact with endo-/lysosomal membranes, which is critical for the light-induced endo-/lysosomal escape of DPc-TPMs ( Fig. 1c ). Subcellular distribution of DPc was observed in HeLa cells after 6 h of incubation with the polyplexes (DPc/Asp(DET)=1) using super-resolution microscopy (structured illumination microscopy; this technique provides better spatial resolution than conventional light microscopy, thereby distinguishing between the lysosomal membrane and the interior of the lysosome more clearly) ( Fig. 4a ). Cy3-labelled pDNA (red) was found inside lysosomes, the membranes of which were visualized using Lamp1-green fluorescent protein (GFP) (green). DPc (blue) was localized on lysosomal membranes and in the lysosomes, indicating that DPc interacts with the lysosomal membranes, presumably after its release from DPc-TPMs in the endo-/lysosomal compartments, as schematically shown in Fig. 4b . 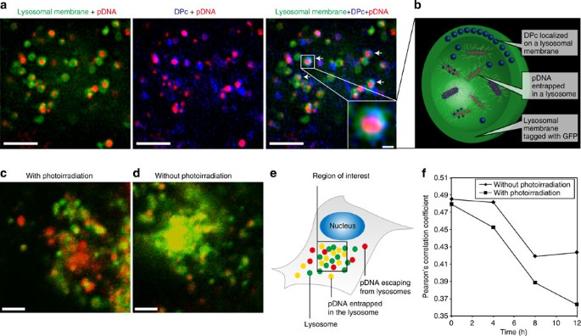Figure 4: The subcellular distribution of DPc-TPMs. (a) Super-resolution microscopic imaging of GFP–lysosomal membranes (green), Cy3-labelled pDNA (red) and DPc (blue). HeLa cells were incubated with DPc-TPMs (DPc/Asp(DET)=1) for 6 h and then fixed. White arrows indicate the colocalization of lysosomal membranes and DPc. Original magnification, × 100. Before selecting this representative image, 18 images (47.58 μm × 47.48 μm (1,904 pixels × 1,900 pixels) × 18 images) were studied. Scale bar, 2 μm (magnified image, 200 nm). (b) Schematic view of the assumed localization of DPc and pDNA in the lysosomal compartment. (c) Confocal imaging of the subcellular distribution of the micelles 15.5 h after photoirradiation. HeLa cells were incubated with DPc-TPMs for 6 h, followed by medium replacement and photoirradiation at a fluence of 2 J cm−2. The image was captured 15.5 h after photoirradiation. Lysosomal membranes were tagged with GFP (green). Cy3-labelled pDNA is shown in red. Original magnification, × 63. This representative image was selected from nine images (134.82 μm × 134.82 μm (1,024 pixels × 1,024 pixels) × 9 images). Scale bar, 2 μm. (d) Confocal imaging of the subcellular distribution of DPc-TPMs without photoirradiation. HeLa cells were incubated with DPc-TPMs at the DPc/Asp(DET) ratio of 1 for 6 h, followed by medium replacement. The image was captured 15.5 h after medium replacement. Original magnification, × 63. This representative image was selected from nine images (134.82 μm × 134.82 μm (1,024 pixels × 1,024 pixels) × 9 images). Scale bar, 2 μm. (e) A schematic diagram used to explain the results shown inc,d. (f) Quantification of Pearson's correlation coefficient between lysosomes–GFP and Cy3-labelled pDNA. The indicated time point indicates the elapsed time after the start of the movie acquisition. Figure 4: The subcellular distribution of DPc-TPMs. ( a ) Super-resolution microscopic imaging of GFP–lysosomal membranes (green), Cy3-labelled pDNA (red) and DPc (blue). HeLa cells were incubated with DPc-TPMs (DPc/Asp(DET)=1) for 6 h and then fixed. White arrows indicate the colocalization of lysosomal membranes and DPc. Original magnification, × 100. Before selecting this representative image, 18 images (47.58 μm × 47.48 μm (1,904 pixels × 1,900 pixels) × 18 images) were studied. Scale bar, 2 μm (magnified image, 200 nm). ( b ) Schematic view of the assumed localization of DPc and pDNA in the lysosomal compartment. ( c ) Confocal imaging of the subcellular distribution of the micelles 15.5 h after photoirradiation. HeLa cells were incubated with DPc-TPMs for 6 h, followed by medium replacement and photoirradiation at a fluence of 2 J cm −2 . The image was captured 15.5 h after photoirradiation. Lysosomal membranes were tagged with GFP (green). Cy3-labelled pDNA is shown in red. Original magnification, × 63. This representative image was selected from nine images (134.82 μm × 134.82 μm (1,024 pixels × 1,024 pixels) × 9 images). Scale bar, 2 μm. ( d ) Confocal imaging of the subcellular distribution of DPc-TPMs without photoirradiation. HeLa cells were incubated with DPc-TPMs at the DPc/Asp(DET) ratio of 1 for 6 h, followed by medium replacement. The image was captured 15.5 h after medium replacement. Original magnification, × 63. This representative image was selected from nine images (134.82 μm × 134.82 μm (1,024 pixels × 1,024 pixels) × 9 images). Scale bar, 2 μm. ( e ) A schematic diagram used to explain the results shown in c , d . ( f ) Quantification of Pearson's correlation coefficient between lysosomes–GFP and Cy3-labelled pDNA. The indicated time point indicates the elapsed time after the start of the movie acquisition. Full size image Upon photoirradiation, DPc localized on lysosomal membranes is expected to disrupt the membrane structures via ROS production, leading to light-selective endo-/lysosomal escape of pDNA into the cytoplasm. This dynamic process was monitored using CLSM ( Fig. 4c–e and Supplementary Movies 1–5 ). After 6 h of incubation with DPc-TPMs, HeLa cells were photoirradiated at a fluence of 2 J cm −2 (halogen lamp, 400–700 nm), and movie acquisition was started 3.5 h after photoirradiation. Initially, most Cy3-labelled pDNA was entrapped in lysosomes. However, 4 h later, some pDNA appeared to leak into the cytoplasm ( Supplementary Movies 1–3 ). Twelve hours after the start of movie acquisition, pDNA became prominent outside the lysosomes, as seen from the clear red fluorescence in Fig. 4c and in Supplementary Movies 1–3 . By contrast, without photoirradiation, such distinctive pDNA translocation was not observed ( Fig. 4d and Supplementary Movies 4 and 5 ). We quantified the colocalization between the lysosomes and pDNA using Pearson’s correlation coefficient (PCC) ( Fig. 4f ). At the start of data acquisition, the PCC value was 0.485 for the non-photoirradiated cells and 0.479 for the photoirradiated cells. The PCC value of the photoirradiated cells then steadily decreased and finally reached 0.363 at 12 h, whereas that of the non-photoirradiated cells only decreased to 0.423. These results are consistent with the PCI-mediated endo-/lysosomal escape of DPc-TPMs. Light-induced endo-/lysosomal escape led to photoenhanced transfection of firefly luciferase ( Fig. 5a ). In the absence of DPc (DPc/Asp(DET)=0), gene expression of the three-layered polyplex micelles was not altered by photoirradiation. However, DPc-TPMs at DPc/Asp(DET) ratios of 1 and 2 resulted in ∼ 44- and 88-fold higher gene expression, respectively, than the polyplex micelle (DPc/Asp(DET)=0), following photoirradiation. By contrast, diblock-TPMs (pDNA/PEG-PLys/DPc) exhibited apparently lower gene expression than DPc-TPMs, regardless of DPc and photoirradiation. DPc-TPMs also achieved photochemically enhanced gene transfer in HCT 116 cells ( Supplementary Fig. 11 and Supplementary Methods ). DPc-TPMs (DPc/Asp(DET)=1 and 2) significantly increased gene expression in a light-induced manner, whereas diblock-TPMs did not accomplish such distinct photochemical enhancement. These results strongly suggest that the three-layered structure of DPc-TPM is critical for light-selective gene transfection. 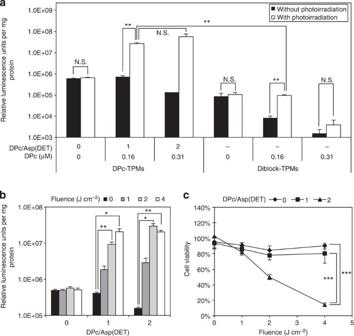Figure 5:In vitrotransfection efficiency and cytotoxicity to HeLa cells. (a) The effect of photoirradiation on the transfection efficiency of DPc-TPMs and diblock-TPMs at DPc concentrations equivalent to DPc/Asp(DET) ratios of 0–2 in DPc-TPMs. Photoirradiation was performed 6 h after incubation with each sample, followed by 40 h post incubation in fresh medium and a subsequent luciferase assay. (b) The effect of photoirradiation fluence on the transfection efficiency of DPc-TPMs at various DPc/Asp(DET) ratios. The same experimental conditions as inawere applied. The results are expressed as means±s.e.m. (n=4). *P<0.05, **P<0.01 (t-test). (c) The cytotoxicity of DPc-TPMs. HeLa cells were incubated with DPc-TPMs for 6 h. The cells were washed with PBS and incubated in fresh medium, followed by photoirradiation with a fluence of 1, 2 or 4 J cm−2and a further 40 h of incubation. For non-photoirradiated cells (0 J cm−2), cells were incubated for 40 h in fresh medium after 6 h of incubation with DPc-TPMs and subsequent washing with PBS. Cell viability was then evaluated using an MTT assay. The results are expressed as means±s.d. (n=8 for 0 J cm−2andn=4 for 1, 2 and 4 J cm−2). ***P<0.000001 (two-way analysis of variance with the Fisher's least significant difference). Figure 5: In vitro transfection efficiency and cytotoxicity to HeLa cells. ( a ) The effect of photoirradiation on the transfection efficiency of DPc-TPMs and diblock-TPMs at DPc concentrations equivalent to DPc/Asp(DET) ratios of 0–2 in DPc-TPMs. Photoirradiation was performed 6 h after incubation with each sample, followed by 40 h post incubation in fresh medium and a subsequent luciferase assay. ( b ) The effect of photoirradiation fluence on the transfection efficiency of DPc-TPMs at various DPc/Asp(DET) ratios. The same experimental conditions as in a were applied. The results are expressed as means±s.e.m. ( n =4). * P <0.05, ** P <0.01 ( t -test). ( c ) The cytotoxicity of DPc-TPMs. HeLa cells were incubated with DPc-TPMs for 6 h. The cells were washed with PBS and incubated in fresh medium, followed by photoirradiation with a fluence of 1, 2 or 4 J cm −2 and a further 40 h of incubation. For non-photoirradiated cells (0 J cm −2 ), cells were incubated for 40 h in fresh medium after 6 h of incubation with DPc-TPMs and subsequent washing with PBS. Cell viability was then evaluated using an MTT assay. The results are expressed as means±s.d. ( n =8 for 0 J cm −2 and n =4 for 1, 2 and 4 J cm −2 ). *** P <0.000001 (two-way analysis of variance with the Fisher's least significant difference). Full size image The effects of photoirradiation fluence on light-induced transfection efficiency and photocytotoxicity in HeLa cells are shown in Fig. 5b and c , respectively. The three-layered polyplex micelle (DPc/Asp(DET)=0) did not affect transfection activity and cytotoxicity upon photoirradiation. DPc-TPMs at DPc/Asp(DET) ratios of 1 and 2 displayed fluence-dependent transfection efficiency, achieving >100-fold increases in light-selective transfection efficiency. With respect to photocytotoxicity, DPc-TPMs at a DPc/Asp(DET) ratio of 2 reduced cell viability with increased fluence. Excess DPc might photochemically damage organelles such as mitochondria or the endoplasmic reticulum after endo-/lysosomal escape [24] . However, DPc-TPMs at a DPc/Asp(DET) ratio of 1 achieved remarkable gene transfer in proportion to fluence without compromising cell viability. This non-cytotoxic PCI effect can be explained by multistep DPc and pDNA delivery: DPc delivery to the endo-/lysosomal membranes to modulate intracellular localization and pDNA delivery to the nucleus to exert gene expression ( Fig. 1c ). In vivo activity of DPc-TPMs The potential of DPc-TPMs to act as light-responsive systemic gene nanocarriers was examined by transfecting a reporter gene (a variant of a yellow fluorescent protein, Venus) into a subcutaneous HeLa tumour in a mouse. We intravenously injected DPc-TPMs at the DPc/Asp(DET) ratio of 1 and photoirradiated the tumour with a semiconductor laser (680 nm, 12 J cm −2 ) 24 h after systemic administration. The tumour was excised 3 days after photoirradiation, and Venus expression was observed using CLSM ( Fig. 6 ). The non-photoirradiated tumour did not show distinct Venus expression (green) ( Fig. 6b ), whereas the photoirradiated tumour did show Venus expression ( Fig. 6c ). Venus fluorescence was quantified from the obtained CLSM images ( Fig. 6d ); the photoirradiated tumour exhibited ∼ 4.4-fold higher fluorescence than the non-photoirradiated tumour. Interestingly, DPc-TPMs also accumulated in highly vascularized organs such as lung, liver, spleen and kidney, resulting in weak gene expression in those organs ( Supplementary Fig. 12 and Supplementary Methods ). However, Venus fluorescence intensity in these organs was significantly lower than that in the photoirradiated tumours ( P <0.01 for lung, P <0.01 for liver and P <0.05 for kidney ( t -test)). The selective gene expression in the tumour is consistent with the PCI function of DPc-TPMs, as demonstrated in Fig. 5 , in which DPc-TPMs exerted distinct gene expression only in the presence of photoirradiation. We also confirmed PCI-mediated gene transfer after systemic administration using a subcutaneous HCT 116 tumour in a mouse ( Supplementary Fig. 13 and Supplementary Methods ). Photoirradiation (30 J cm −2 ) to HCT 116 tumours 24 h after systemic administration of DPc-TPMs resulted in photochemically enhanced Venus expression. The photoirradiated tumour exhibited ∼ 6.0-fold higher Venus fluorescence than the non-photoirradiated tumour. To our knowledge, these experiments are the first successful demonstrations of PCI-mediated gene transfection after systemic administration. 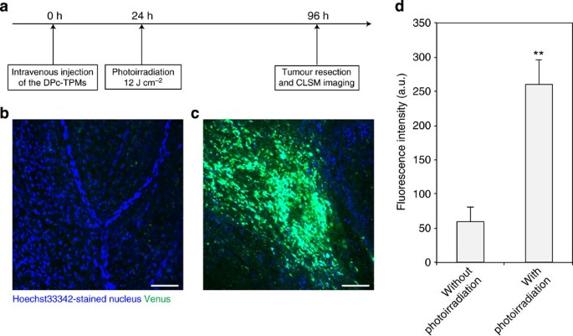Figure 6:In vivotransfection into a subcutaneous HeLa tumour model. (a) A scheme showingin vivotransfection. (b,c)Ex vivoCLSM images of the tumours (b) without photoirradiation and (c) with photoirradiation. A Hoechst 33342-stained nucleus and Venus fluorescence are shown in blue and green, respectively. Scale bars, 100 μm. (d) The Venus fluorescence intensity was quantified from the images after subtraction of the background intensity. The results are expressed as means±s.e.m. (n=5 mice for tumours without photoirradiation andn=6 mice for tumours with photoirradiation). **P<0.01 (t-test). Figure 6: In vivo transfection into a subcutaneous HeLa tumour model. ( a ) A scheme showing in vivo transfection. ( b , c ) Ex vivo CLSM images of the tumours ( b ) without photoirradiation and ( c ) with photoirradiation. A Hoechst 33342-stained nucleus and Venus fluorescence are shown in blue and green, respectively. Scale bars, 100 μm. ( d ) The Venus fluorescence intensity was quantified from the images after subtraction of the background intensity. The results are expressed as means±s.e.m. ( n =5 mice for tumours without photoirradiation and n =6 mice for tumours with photoirradiation). ** P <0.01 ( t -test). Full size image Previous studies have revealed the validity of PCI as a method for the cytoplasmic delivery of anticancer drugs, genes, small interfering RNAs and immunotoxins [13] , [14] , [15] , [16] , [25] , [26] , [27] . PCI is notably successful in anticancer drug delivery; the use of PCI in combination with bleomycin is now in phase II clinical studies. However, in vivo application of PCI with nucleic acid compounds, including pDNA, has remained limited because the development of nanocarriers is a prerequisite for their delivery. We previously developed a light-responsive nanocarrier and succeeded in light-selective gene transfection after local administration [23] ; however, the nanocarrier could be further improved for use in systemic applications. In this context, polymeric micellar structures offer great potential for systemic applications because polymeric micelles have been widely studied as systemically injectable nanocarrier platforms, and their therapeutic efficacy has been demonstrated [28] , [29] , [30] , [31] , [32] , [33] . The core compartment encapsulates therapeutic pDNA and protects it from enzymatic degradation; the shell compartment inhibits unfavourable interactions with biological components, yielding prolonged circulation times. Owing to these characteristics, the polyplex micelles can accumulate within highly vascularized tumours and exert therapeutic efficacy. In this study, to mount PCI function into the polyplex micelle, we synthesized PEG-PAsp(DET)-PLys, thereby enabling the construction of DPc-TPMs containing an intermediate layer encapsulating DPc to achieve systemic light-selective gene transfer. In DPc-TPMs, pDNA exhibited rod-shaped structures ( Fig. 2 ) consistent with our previously reported scheme in which pDNA was regularly folded through the interaction with PEG-polycation block copolymers [34] . The pDNA in the DPc-TPMs then exhibited unique morphological changes depending on the DPc/Asp(DET) ratio. As schematically illustrated in Supplementary Fig. 14 , these morphological changes may be explained by considering electrostatic repulsion and ion osmotic pressure in the intermediate compartment. DPc incorporation neutralizes the charge in PAsp(DET), eventually reducing electrostatic repulsion and releasing small counterions to decrease the ion osmotic pressure in the intermediate compartment, thereby leading the polyplex rod to contract to compensate for the interfacial free energy. Further increase in the DPc fraction in the compartment beyond the charge stoichiometry, in turn, generates electrostatic repulsion and increases the ion osmotic pressure, thus extending the polyplex rod. This scheme is in good agreement with the zeta potential profile presented in Supplementary Fig. 5 . Incorporation of DPc into the intermediate layer led to stable pDNA packaging ( Fig. 3 ). In the random-TPM, DPc and pDNA form polyion complexes randomly with PAsp(DET) and PLys, thereby hampering pDNA condensation and placing DPc and pDNA close to each other. However, DPc-TPMs were constructed through the sequential assembly of pDNA, PEG-PAsp(DET)-PLys and DPc; in this way, DPc and pDNA were accommodated into segregated compartments, stably packaging the pDNA. This structural difference also affected the level of pDNA oxidative damage ( Supplementary Fig. 9 ). According to a previous study [35] , the lifetime of singlet oxygen (considered to be a major product of an activated PS) is <0.1 ms, and the distance that singlet oxygen can travel in the cell is correspondingly estimated to be 10–20 nm. Considering the length of the PAsp(DET) strand, the distance between DPc and pDNA in DPc-TPMs is estimated to be <20 nm. Thus, singlet oxygen produced in the intermediate layer can reach pDNA in the core compartment. Consistent with these theoretical values, we observed some damage to pDNA. However, because singlet oxygen decays exponentially with time, longer distances between DPc and pDNA are expected to considerably alleviate pDNA damage. Indeed, pDNA in DPc-TPMs exhibited substantially less damage than that in random-TPMs. In addition, in the endo-/lysosomes studied, DPc was released from the DPc-TPMs and localized to lysosomal membranes ( Fig. 4 ), decreasing the amount of DPc in the DPc-TPMs. We confirmed that the decreased amount of DPc reduced the level of oxidative damage ( Supplementary Fig. 15 ). DPc-TPMs (DPc/Asp(DET)=2) exhibited 69% of the original fluorescence intensity of supercoiled pDNA after photoirradiation at 2 J cm −2 ( Supplementary Fig. 9 ); by contrast, DPc-TPMs (DPc/Asp(DET)=1 and 0.5) exhibited 78% and 85% of the original fluorescence intensity of supercoiled pDNA after photoirradiation at 2 J cm −2 , respectively ( Supplementary Fig. 15 ). Thus, the oxidative damage to pDNA experienced during the PCI process inside the cell might be lower than that estimated in this model experiment ( Supplementary Fig. 9 ). In our in vitro study, DPc-TPMs exhibited multistep DPc and pDNA delivery. DPc was delivered to the lysosomal membranes in response to the acidic conditions prevailing in the lysosome, thereby inducing a PCI effect ( Fig. 4 ); pDNA was transferred to the nucleus at high transfection efficiency ( Fig. 5 and Supplementary Fig. 11 ). In our in vivo study, more importantly, DPc-TPMs demonstrated light-selective transfection in subcutaneous HeLa and HCT 116 tumours after systemic administration, as shown in Fig. 6 and Supplementary Fig. 13 . Although many previous studies have reported systemic nanocarriers for gene delivery into tumours, these nanocarriers inevitably accumulate into highly vascularized normal organs, including lung, liver, spleen and kidney, resulting in non-specific gene expression in these organs. In this regard, spatiotemporal control by PCI is a promising approach for selective gene transfer after systemic administration. Indeed, owing to PCI function in the intermediate layer ( Figs 4 and 5 and Supplementary Fig. 11 ), the DPc-TPMs accomplished light-selective gene expression in the tumour even though some accumulation was observed in normal organs ( Supplementary Fig. 12 ). These results strongly demonstrate the benefit of combining PCI with systemic site-specific gene transduction. The three-layered micelle concept can be extended to create a universal platform for multistep delivery of therapeutic agents in a spatiotemporally controlled manner. Nanocarrier platforms integrated with such multiple functions offer a promising strategy for overcoming biological barriers (for example, limited extravasation, poor tissue penetration and drug resistance) to treat intractable diseases. Synthesis of PEG-PAsp(DET)-PLys triblock copolymer PEG-PAsp(DET)-PLys triblock copolymer was synthesized as described previously [18] with a minor modification. In brief, as the precursor of PEG-PAsp(DET)-PLys triblock copolymer, PEG- b -poly(β-benzyl-L-aspartate)- b -poly[ ∈ -(benzyloxycarbonyl)-L-lysine] (PEG-PBLA-PLys(Z)) was synthesized by the sequential ring-opening polymerization of BLA N -carboxyanhydride and Lys(Z) N -caryboxyanhydride, initiated by α-methoxy-ω-amino-PEG as described previously [18] . The molecular weight distribution (Mw/Mn) of PEG-PBLA-PLys(Z) was determined as 1.05 by gel permeation chromatography, using TOSOH HLC-8220 equipped with TSKgel columns (Super AW4000 and Super AW3000 × 2) and an internal refractive index detector (Tosoh Corporation, Tokyo, Japan). N -methyl-2-pyrrolidone containing 50 mM lithium bromide was used as an eluent (flow rate: 0.3 ml min −1 ; temperature: 40 °C). The amino group of the N-terminal of PEG-PBLA-PLys(Z) was then acetylated using acetic anhydride in dichloromethane. Next, PEG-PBLA-PLys(Z) was lyophilized with benzene and dissolved in N -methyl-2-pyrrolidone, after which aminolysis was conducted using diethylenetriamine (50 eq. to the benzyl groups in PBLA) at 0 °C for 1 h. After aminolysis, the solution was neutralized with hydrochloric acid (HCl), dialysed in 0.01 M HCl and lyophilized, followed by microfiltration in water through a 0.02-μm pore-size filter; the residue was then lyophilized. The resulting polymer was dissolved in trifluoroacetic acid, and hydrogen bromide (30% in acetic acid) was added to deprotect the Z groups in the PLys(Z) segment. After 1 h of stirring, the solution was added dropwise into diethyl ether. The resulting precipitate was filtered, dissolved in water, dialysed against 0.01 M HCl and lyophilized to obtain the hydrochloride salt form of PEG-PAsp(DET)-PLys. The DPs of PAsp(DET) and PLys were confirmed using 1 H NMR using a JEOL EX300 spectrometer (JEOL Ltd, Tokyo, Japan). Synthesis of DPc DPc was synthesized according to a previously reported method [36] . First, dendritic phthalonitrile was obtained by an alkali-mediated coupling reaction of 4-nitrophthalonitrile and a second generation of dendritic phenol. To obtain DPc, the dendritic phthalonitrile was treated with Zn(OAc) 2 and 1,8-diazabicyclo[5,4,0]undec-7-ene in n -pentanol, followed by treatment with NaOH in a mixed tetrahydrofuran/H 2 O solution. Preparation of DPc-TPMs PEG-PAsp(DET)-PLys and pDNA were separately dissolved in 10 mM HEPES (2-[4-(2-hydroxyethyl)-1-piperazinyl]ethanesulphonic acid) buffer (pH 7.3). The polymer solution was then added to a solution of pDNA at a fixed concentration (50 μg ml −1 ) to form polyplex micelles at a Lys/pDNA ratio of 1. The final concentration of pDNA was fixed at 33.3 μg ml −1 for all experiments, except for the 1 H NMR, ultracentrifuge, TEM, FRET and in vivo experiments. The pDNA/PEG-PAsp(DET)-PLys polyplex micelles were maintained at 4 °C for at least 10 min, after which the DPc solution (in 10 mM HEPES buffer (pH 7.3)) was added at varying DPc/Asp(DET) ratios; the final pDNA concentration was fixed at 30.3 μg ml −1 . The protonation degrees of Lys and Asp(DET) units were estimated at pH 7.3 as 1.0 and 0.5, respectively, based on the potentiometric titration results reported in our previous study [19] . 1 H NMR measurement Deuterated 10 mM phosphate buffer containing 150 mM NaCl (pH 7.4) was used to prepare the pDNA/PEG-PAsp(DET)-PLys polyplex micelles. pDNA/PEG-PAsp(DET)-PLys polyplex micelles were prepared at a fixed pDNA concentration (166.7 μg ml −1 ). The measurements of PEG-PAsp(DET)-PLys copolymer (5 mg ml −1 ) and the polyplex micelles were accumulated 64 and 4,096 times, respectively, at 25 °C using a JEOL EX300 spectrometer (JEOL Ltd). Gel retardation assay pDNA and DPc-TPMs were electrophoresed through a 0.9 wt% agarose gel in TAE buffer (3.3 mM Tris-acetic acid (pH 7.4)+1.7 mM sodium acetate+1 mM EDTA/2Na). pDNAs were then stained using 0.5 mg l −1 ethidium bromide in distilled water. Ultracentrifugation pDNA/PEG-PAsp(DET)-PLys polyplex micelles were prepared at the pDNA concentration of 200 μg ml −1 . DPc was then added to the polyplex micelle solution. The final concentration of pDNA was fixed at 182 μg ml −1 . The DPc-TPM solution was centrifuged at 62,800 g for 2 h (4 °C) to sediment the polyplex micelles using an ultracentrifuge (Optima TLX, Beckman Coulter, Inc., Fullerton, CA, USA). The supernatant was carefully transferred, and the absorption of the supernatant at 670 nm was measured to quantify the amount of DPc not incorporated into the polyplex micelle. Size and zeta potential of the prepared DPc-TPMs The size of DPc-TPMs was evaluated by dynamic light scattering at 25 °C using a Zetasizer Nano Series (Malvern Instruments Ltd, Worcestershire, UK) instrument equipped with a laser operating at 532 nm and using a detection angle of 173°. The zeta potential was measured by laser Doppler electrophoresis using a Zetasizer Nano Series instrument equipped with a He–Ne laser (633 nm). Transmission electron microscopy DPc-TPMs were prepared at the pDNA concentration of 15.2 μg ml −1 . DPc-TPMs at various DPc/Asp(DET) ratios were stained with uranyl acetate and observed using an H-7000 electron microscope (Hitachi Ltd., Tokyo, Japan). The lengths of 100 polyplex micelles were measured using ImageJ software (National Institutes of Health, Bethesda, MD, USA). FRET experiments pDNA was labelled with fluorescein and Cy3 using Label IT Tracker Subcellular Nucleic Acid Localization Kits as described previously [22] . Fluorescein and Cy3 were used as the donor–acceptor pair. To form pDNA/PEG-PAsp(DET)-PLys/DPc (DPc-TPM), a solution of PEG-PAsp(DET)-PLys was added to the fluorescein-Cy3-labelled pDNA solution at a fixed concentration (150 μg ml −1 ) at the Lys/pDNA ratio of 1, after which a DPc solution was added at various DPc/Asp(DET) ratios. The pDNA concentration was fixed at 90.9 μg ml −1 in each sample. pDNA/PEG-PLys/DPc diblock-TPMs were prepared in the same manner at a Lys/pDNA ratio of 1.5. To form (pDNA+DPc)/PEG-PAsp(DET)-PLys (random-TPM), pDNA and DPc were mixed at a fixed pDNA concentration (130 μg ml −1 ), after which a solution of PEG-PAsp(DET)-PLys was added at varying DPc/Asp(DET) ratios. The fluorescence intensity of each sample was measured using a ND-3300 spectrofluorometer (NanoDrop Technologies, Wilmington, DE, USA) with excitation at 470±10 nm. The ratio of fluorescence intensity at 526 nm to that at 569 nm (fluorescein/Cy3) was calculated as a FRET indicator. Photostability of incorporated pDNA Forty microlitres of the DPc-TPM solution and 40 μl of the random-TPM solution were photoirradiated using a 300-W halogen lamp (fluence rate, 3.0 mW cm −2 ) equipped with a band filter (400–700 nm), after which 40 μl of sodium dextran sulphate solution (100 mg ml −1 ) in 10 mM HEPES buffer (pH 7.3) was added to dissociate the polyplex micelles. The samples were then electrophoresed through a 0.9 wt% agarose gel (running buffer: 3.3 mM Tris-acetic acid (pH 7.4)+1.7 mM sodium acetate+1 mM EDTA/2Na). After electrophoresis, pDNAs in the gel were stained using SYBR Green I. The SYBR Green I fluorescence of pDNA was quantified using a Molecular Imager FX Pro (Bio-Rad Laboratories Inc., Hercules, CA, USA) instrument. Super-resolution imaging of subcellular distributions The human cervical carcinoma cell line HeLa was obtained from the cell bank of the RIKEN Bioresource Center, Ibaraki, Japan. The cells were grown in DMEM supplemented with 50 μg ml −1 penicillin/streptomycin and 10% (v/v) FBS in a 5% CO 2 /air incubator at 37 °C. pDNA was labelled with Cy3 using the Label IT Tracker Subcellular Nucleic Acid Localization Kit according to the manufacturer’s protocol. In total, 20,000 HeLa cells were seeded on a 35-mm glass-based dish and incubated overnight. After replacing the medium with 1 ml of fresh medium, CellLight Lysosomes–GFP was applied. After 3 days of incubation with CellLight Lysosomes–GFP and medium replacement, a DPc-TPM solution (DPc/Asp(DET)=1) containing 3 μg of Cy3-labelled pDNA was applied to the cells. After 6 h of incubation, the medium was removed; the cells were then fixed with 4% paraformaldehyde in PBS (phosphate-buffered saline) and observed under an ELYRA PS.1-structured illumination microscope, (Carl Zeiss Inc., Oberkochen, Germany). GFP, Cy3 and DPc were excited using laser light at 488 nm, 561 nm and 642 nm, respectively. Confocal imaging of PCI In total, 20,000 HeLa cells were seeded on a 35-mm glass-based dish and incubated overnight. After replacing the medium, CellLight Lysosomes–GFP was applied. After 3 days of incubation with CellLight Lysosomes–GFP and medium replacement, a DPc-TPM solution (DPc/Asp(DET)=1) containing 3 μg of Cy3-labelled pDNA was applied to the cells. After 6 h of incubation, the medium was replaced, and the cells were photoirradiated at a fluence of 2 J cm −2 using a 300-W halogen lamp (fluence rate, 3.0 mW cm −2 ) equipped with a band filter (400–700 nm). The photoirradiated cells were then incubated for an additional 3.5 h, after which the subcellular distribution of DPc-TPMs was observed using a CLSM, LSM 780 (Carl Zeiss Inc.) instrument, equipped with an incubator (Tokai Hit Co., Ltd, Shizuoka, Japan), thereby maintaining the temperature at 36.5 °C under a humidified atmosphere containing 5% CO 2 /air. GFP and Cy3 were excited with laser light at 488 nm and 561 nm, respectively. The emission wavelengths of GFP and Cy3 were set to 489–551 nm and 568–629 nm, respectively. The acquisition interval used in the time-series imaging was set to 15 min. The data obtained in the time-series imaging were analysed using Imaris software (Bitplane, Zurich, Switzerland) to estimate the PCC between GFP and Cy3. In vitro transfection and cytotoxicity assays In total, 10,000 HeLa cells per well were plated on 24-well plates 24 h before transfection. The cells were then incubated with DPc-TPMs or diblock-TPMs containing 1 μg of pDNA. After 6 h of incubation at 37 °C, the cells were washed with PBS, after which the medium was replaced. The cells were then irradiated using a 300-W halogen lamp (fluence rate, 3.0 mW cm −2 ) equipped with a band filter (400–700 nm). After an additional 40 h of incubation following photoirradiation, the cells were washed with PBS and lysed with 200 μl of Cell-LyEX 1 per well. Luciferase gene expression was evaluated using LB940 (Berthold Technologies, Bad Wildbad, Germany) or Glomax (Promega). The amount of protein in each well was determined using a Micro BCA Protein Assay Reagent Kit. Cell viability was evaluated using the 3-(4,5-dimethylthiazol-2-yl)-2,5-diphenyltetrazolium bromide (MTT) assay. In vivo transfection Female 5-week-old C.B-17 severe combined immunodeficiency (SCID) mice and female 5-week-old BALB/c nude mice were obtained from Charles River Laboratories Japan Inc. (Kanagawa, Japan). All animal experiments were performed in accordance with the Guidelines for the Care and Use of Laboratory Animals as stated by the University of Tokyo. HeLa cells were inoculated into a C.B-17 SCID mouse. The resulting tumours were then subcutaneously transplanted into BALB/c nude mice. When the tumour size reached ∼ 100 mm 3 , 220 μl of a DPc-TPM solution containing pDNA encoding Venus at a DPc/Asp(DET) ratio of 1 (182 μg ml −1 of pDNA) was intravenously injected. Twenty-four hours after injection, the mice were anesthetized with isoflurane (Abbott Japan Co., Ltd, Tokyo, Japan), and the tumour sites were irradiated with a diode laser at 680 nm (maximum output: 2 W, numerical aperture: 0.22, B&W TEK, Newark, DE, USA) at a dose of 12 J cm −2 . Three days after photoirradiation, Hoechst 33342 (5 mg kg −1 in PBS) was intravenously injected to stain the nuclei. The tumours were then excised and observed using a Nikon A1R CLSM (Nikon Corp., Tokyo, Japan). Hoechst 33342 and Venus were excited with laser light at 405 nm and 488 nm, respectively. The emission wavelengths of Hoechst 33342 and Venus were set to 425–475 nm and 500–550 nm, respectively. Image processing was performed using Nikon NIS Elements software (Nikon Corp.). Venus fluorescence was quantified by subtraction of the background intensity from the mean fluorescence intensity of each image. The background intensity was obtained from the image of a tumour excised from a non-treated tumour-bearing mouse. The average Venus fluorescence intensity in each mouse was calculated from eight images, and the mean fluorescent intensities and standard errors were calculated from five mice for tumours without photoirradiation, and from six mice for tumours with photoirradiation. How to cite this article: Nomoto, T. et al. Three-layered polyplex micelle as a multifunctional nanocarrier platform for light-induced systemic gene transfer. Nat. Commun. 5:3545 doi: 10.1038/ncomms4545 (2014).